p85α recruitment by the CD300f phosphatidylserine receptor mediates apoptotic cell clearance required for autoimmunity suppression Apoptotic cell (AC) clearance is essential for immune homeostasis. Here we show that mouse CD300f (CLM-1) recognizes outer membrane-exposed phosphatidylserine, and regulates the phagocytosis of ACs. CD300f accumulates in phagocytic cups at AC contact sites. Phosphorylation within CD300f cytoplasmic tail tyrosine-based motifs initiates signals that positively or negatively regulate AC phagocytosis. Y276 phosphorylation is necessary for enhanced CD300f-mediated phagocytosis through the recruitment of the p85α regulatory subunit of phosphatidylinositol-3-kinase (PI3K). CD300f-PI3K association leads to activation of downstream Rac/Cdc42 GTPase and mediates changes of F-actin that drive AC engulfment. Importantly, primary macrophages from CD300f-deficient mice have impaired phagocytosis of ACs. The biological consequence of CD300f deficiency is predisposition to autoimmune disease development, as FcγRIIB-deficient mice develop a systemic lupus erythematosus-like disease at a markedly accelerated rate if CD300f is absent. In this report we identify the mechanism and role of CD300f in AC phagocytosis and maintenance of immune homeostasis. Apoptosis is an essential element of many physiological and pathological processes [1] , [2] . The rapid and efficient removal of apoptotic cells (ACs) prevents the generation of secondary necrosis and the release of potentially toxic or immunogenic components from necrotic cells, reducing the likelihood of inflammatory and autoimmune responses [3] , [4] , [5] , [6] , [7] . Phagocytosis is the major means of clearing AC, and is mediated by neighbouring cells, or professional phagocytes, such as macrophages and immature dendritic cells [7] , [8] , [9] , [10] , [11] . ACs are recognized through their display of characteristic cell surface molecules, known as ‘eat-me’ signals [6] , [7] , [8] . The best-known ‘eat-me’ signal for phagocytes is phosphatidylserine (PS), which serves as a common AC recognition cue for multiple phagocytic receptors [7] , [8] , [12] , [13] . Some receptors bind PS directly, for example, Tim4 (ref. 14 ), stabilins [15] , [16] or BAI1 (ref. 17 ). Other receptors recognize PS via soluble PS-binding bridging molecules, for instance MFG-E8 or Gas6 (refs 6 , 7 , 8 ). Recently, we showed that CD300 family members CD300a [18] and mouse CD300f (CLM-1) [19] also bind PS, and their overexpression in cell lines regulates AC phagocytosis. The signalling mechanism underlying the phagocytosis by opsonin receptor (Fc and complement) targets, usually bacteria or RBCs, has been somewhat described [8] , [20] . Although signalling pathways including CrkII/DOCK180/ELMO/Rac1, GULP/Rac1, GRK6/GIT1/Rac1 and Vav1/Rho GTPase (Rac1, Cdc42 or RhoA) have been shown to regulate actin polymerization during AC phagocytosis by nematode and mammalian phagocytes [17] , [21] , [22] , [23] , [24] , [25] , [26] , [27] , much less, compared with opsonin receptors, is known about the signalling mechanism(s) governing the phagocytosis of AC mediated by ‘eat-me’ signals, like PS. The CD300 family consists of both activating and inhibitory members [28] . The activating members have short intracellular tails and gain activation potential by association with adaptor proteins (e.g., DAP12) containing immunoreceptor tyrosine-based activation motifs. The inhibitory members have intracellular tails containing immunoreceptor tyrosine-based inhibitory motifs. CD300f, expressed on myeloid cells and a subset of B cells, is unique in having both activating and inhibitory motifs in its intracellular tail [28] . Antibody cross-linking of human [29] and mouse [30] , [31] , [32] CD300f has been shown to inhibit or activate several cellular processes. Here we show that CD300f promotes PS-dependent AC phagocytosis by primary macrophages, and CD300f deficiency contributes to the development and pathogenesis of systemic lupus erythematosus in a mouse model. We demonstrate that CD300f works as a tethering and signalling molecule that initiates AC phagocytosis. Upon incubation of phagocytes with AC, the phosphorylation of Y276 mediates the recruitment of the p85α regulatory subunit of phosphatidylinositol-3-kinase (PI3K). This association results in activation of the small GTPase Rac/Cdc42 and leads to actin cytoskeleton rearrangements at the phagocytic cups for efficient phagocytosis. Curiously, CD300f can also generate inhibitory signals that serve to dampen AC phagocytosis. CD300f positively regulates AC phagocytosis by macrophages Our previous data indicated that CD300f could promote AC phagocytosis when overexpressed in a fibroblast cell line [19] . To verify this, we used apoptotic thymocytes labelled with a pH-sensitive dye pHrodo that become flourogenic only if phagocytized [33] . CD300f overexpressing L929 cells were remarkably more efficient at phagocytosis than empty virus-transduced cells ( Fig. 1a,b ). Similar results were obtained with NIH3T3 fibroblast cells ( Supplementary Fig. 1 ). We validated the cell line results using primary alveolar and peritoneal macrophages from Cd300f −/− mice. CD300f-deficient macrophages were half as efficient at AC phagocytosis as macrophages from wt mice ( Fig. 1c–f ). Bone marrow-derived macrophages (BMDM) from Cd300f −/− mice also exhibited impaired phagocytic capability ( Fig. 1g ). Importantly, the effect of CD300f deficiency on phagocytosis was also observed in vivo , as significantly fewer CD300f null peritoneal macrophages had engulfed AC than wt macrophages at 90 min ( Fig. 1h ). Thus, CD300f plays important roles in positively regulating AC phagocytosis in vitro and in vivo. 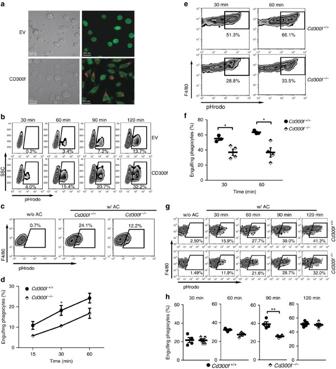Figure 1: CD300f positively regulates the phagocytosis of AC. (a) CFSE-labelled L929 cells (green), transduced with empty virus (EV) or lentivirus encoding CD300f, were mixed with pHrodo-labelled AC at a 1:15 ratio. After 2 h, the cells were mounted on a slide in the pH 8.8 buffer (to quench pHrodo fluorescence signal from non-engulfed AC) and analysed by confocal microscopy. The engulfed pHrodo-labelled ACs are red; the differential interference contrast (DIC) images are shown on the left. Scale bars, 20 μm. (b) L929 cells, transduced with the indicated constructs, were mixed with pHrodo-labelled AC at a 1:3 ratio for the indicated times. Cells were suspended in the pH 8.8 buffer and analysed for the percentage of pHrodo+cells, representing the cells that engulfed AC. (c,d) Primary alveolar cells isolated from threewtorCd300f−/−mice were incubated with pHrodo-labelled AC at a 1:3 ratio for the indicated times (w/AC) or left alone (w/o AC). Cells were stained with anti-mouse F4/80 Ab and analysed for the percentage of F4/80+pHrodo+cells from F4/80-positive population, representing the macrophages that engulfed AC. The plots (c) illustrate the gating strategy used; numbers indicate the percentage of F4/80+pHrodo+cells. The graph (d) shows means±s.e.m. (error bars),n=3. (e,f) Peritoneal cells isolated fromwtorCd300f−/−mice were treated and analysed as inc) with gating on F4/80+CD11b+cells. The plots (e) illustrate the gating strategy used. The graph (f) shows means±s.e.m. (error bars) for threewtand fourCd300f−/−mice; data are representative from three experiments. Asterisks in (d) and (f) indicate statistical significance (*P<0.05, Student’st-test). (g) BMDM fromwtandCd300f−/−mice were mixed with pHrodo-labelled AC and analysed as in (c). The data shows a representative result from three experiments. (h) pHrodo-labelled ACs (1 × 106) were intraperitoneally injected intowtandCd300f−/−mice. At the indicated time points, peritoneal cells were collected, labelled with anti-mouse F4/80 and anti-mouse CD11b Ab and analysed as in (c). The data show means±s.e.m. (error bars) for fourwtandCd300f−/−mice, and are representative of three experiments. Asterisks indicate statistical significance (**P<0.01, Student’st-test). Figure 1: CD300f positively regulates the phagocytosis of AC. ( a ) CFSE-labelled L929 cells (green), transduced with empty virus (EV) or lentivirus encoding CD300f, were mixed with pHrodo-labelled AC at a 1:15 ratio. After 2 h, the cells were mounted on a slide in the pH 8.8 buffer (to quench pHrodo fluorescence signal from non-engulfed AC) and analysed by confocal microscopy. The engulfed pHrodo-labelled ACs are red; the differential interference contrast (DIC) images are shown on the left. Scale bars, 20 μm. ( b ) L929 cells, transduced with the indicated constructs, were mixed with pHrodo-labelled AC at a 1:3 ratio for the indicated times. Cells were suspended in the pH 8.8 buffer and analysed for the percentage of pHrodo + cells, representing the cells that engulfed AC. ( c , d ) Primary alveolar cells isolated from three wt or Cd300f − / − mice were incubated with pHrodo-labelled AC at a 1:3 ratio for the indicated times (w/AC) or left alone (w/o AC). Cells were stained with anti-mouse F4/80 Ab and analysed for the percentage of F4/80 + pHrodo + cells from F4/80-positive population, representing the macrophages that engulfed AC. The plots ( c ) illustrate the gating strategy used; numbers indicate the percentage of F4/80 + pHrodo + cells. The graph ( d ) shows means±s.e.m. (error bars), n =3. ( e , f ) Peritoneal cells isolated from wt or Cd300f − / − mice were treated and analysed as in c ) with gating on F4/80 + CD11b + cells. The plots ( e ) illustrate the gating strategy used. The graph ( f ) shows means±s.e.m. (error bars) for three wt and four Cd300f − / − mice; data are representative from three experiments. Asterisks in ( d ) and ( f ) indicate statistical significance (* P <0.05, Student’s t -test). ( g ) BMDM from wt and Cd300f − / − mice were mixed with pHrodo-labelled AC and analysed as in ( c ). The data shows a representative result from three experiments. ( h ) pHrodo-labelled ACs (1 × 10 6 ) were intraperitoneally injected into wt and Cd300f − / − mice. At the indicated time points, peritoneal cells were collected, labelled with anti-mouse F4/80 and anti-mouse CD11b Ab and analysed as in ( c ). The data show means±s.e.m. (error bars) for four wt and Cd300f − / − mice, and are representative of three experiments. Asterisks indicate statistical significance (** P <0.01, Student’s t -test). Full size image CD300f recognizes PS for regulation of AC phagocytosis Although we identified PS as a ligand for CD300f [19] , the ligand specificity is a matter of continuing debate [34] , [35] . Therefore, we rigorously verified PS recognition by CD300f. Pretreatment of AC with annexin V or MFG-E8, the PS-binding proteins with high affinity [36] , markedly inhibited the promoting effect of CD300f on phagocytosis ( Fig. 2a,b ). Similarly, the addition of liposomes containing PS completely blocked CD300f-mediated phagocytosis, while liposomes containing phosphatidylethanolamine, phosphatidylcholine (PC) or ceramide had no effect ( Fig. 2c ). Liposomes containing phosphatidylglycerol (PG) inhibited phagocytosis by ~50%. Moreover, PS liposome-coated, but not PC-liposome-coated beads were engulfed by CD300f-expressing phagocytes ( Fig. 2d,e ). Furthermore, mutation of the Asp residue at position 117, a putative calcium-binding site, eliminated the ability of CD300f to bind AC and mediate their phagocytosis ( Supplementary Fig. 2 ). These results support the conclusion that CD300f-mediated phagocytosis is due to specific recognition of PS. 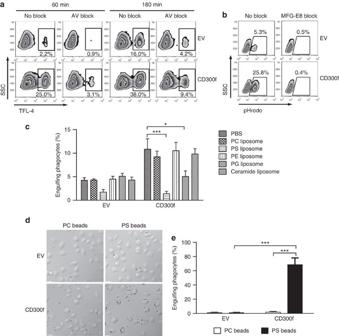Figure 2: Specific recognition of PS is essential for CD300f-mediated phagocytosis of AC. (a) TFL-4 labelled AC were untreated (no block) or were pretreated with 50 μg ml−1recombinant annexin V (AV block) and then mixed with the EV or CD300f-transduced L929 cells at a 3:1 ratio for 1 or 3 h. Following the incubation, the cells were fixed and analysed by flow cytometry. The percentage of L929 cells that phagocytosed AC (TFL-4high) is shown below the gating region. The result shown is representative of two experiments. (b) pHrodo-labelled ACs were untreated (no block) or were pretreated with 20 μg ml−1recombinant MFG-E8 and then mixed with the EV or CD300f-transduced L929 cells at a 3:1 ratio for 1 h. Following the incubation, the cells were fixed and analysed by flow cytometry as forFig. 1b. (c) EV or CD300f-transduced L929 cells were preincubated with the liposomes (10 μM) containing phosphatidylcholine (PC), PS, phosphatidylethanolamine (PE), phosphatidylglycerol (PG) or ceramide for 10 min at 37 °C and then mixed at a 1:2 ratio with pHrodo-labelled AC in the presence of liposomes. After 1 h incubation, the cells were suspended in the pH 8.8 buffer and analysed by flow cytometry for the percentage of L929 cells that engulfed AC. The graph shows means with s.e.m. (error bars) from three experiments. Asterisks indicate statistical significance (*P<0.05, ***P<0.001, Student’st-test). (d,e) PC or PS liposome-coated beads were added to L929 cells transduced with EV or CD300f WT. After 30 min incubation, the cells were washed, fixed and imaged by microscopy. (d) The DIC images show the cells and the liposome-coated beads; the scale bar is 20 μm. (e) The graph represents the means with s.e.m. (error bars) from the analysis of 100 cells from four or five random fields of view. Asterisks indicate statistical significance (***P<0.001, Student’st-test). Figure 2: Specific recognition of PS is essential for CD300f-mediated phagocytosis of AC. ( a ) TFL-4 labelled AC were untreated (no block) or were pretreated with 50 μg ml −1 recombinant annexin V (AV block) and then mixed with the EV or CD300f-transduced L929 cells at a 3:1 ratio for 1 or 3 h. Following the incubation, the cells were fixed and analysed by flow cytometry. The percentage of L929 cells that phagocytosed AC (TFL-4 high ) is shown below the gating region. The result shown is representative of two experiments. ( b ) pHrodo-labelled ACs were untreated (no block) or were pretreated with 20 μg ml −1 recombinant MFG-E8 and then mixed with the EV or CD300f-transduced L929 cells at a 3:1 ratio for 1 h. Following the incubation, the cells were fixed and analysed by flow cytometry as for Fig. 1b . ( c ) EV or CD300f-transduced L929 cells were preincubated with the liposomes (10 μM) containing phosphatidylcholine (PC), PS, phosphatidylethanolamine (PE), phosphatidylglycerol (PG) or ceramide for 10 min at 37 °C and then mixed at a 1:2 ratio with pHrodo-labelled AC in the presence of liposomes. After 1 h incubation, the cells were suspended in the pH 8.8 buffer and analysed by flow cytometry for the percentage of L929 cells that engulfed AC. The graph shows means with s.e.m. (error bars) from three experiments. Asterisks indicate statistical significance (* P <0.05, *** P <0.001, Student’s t -test). ( d , e ) PC or PS liposome-coated beads were added to L929 cells transduced with EV or CD300f WT. After 30 min incubation, the cells were washed, fixed and imaged by microscopy. ( d ) The DIC images show the cells and the liposome-coated beads; the scale bar is 20 μm. ( e ) The graph represents the means with s.e.m. (error bars) from the analysis of 100 cells from four or five random fields of view. Asterisks indicate statistical significance (*** P <0.001, Student’s t -test). Full size image CD300f tail initiates phagocytic signals To determine whether CD300f promotes AC phagocytosis simply through tethering or by initiating signalling, we created a CD300f mutant, lacking the cytoplasmic tail (ΔCT) ( Fig. 3a ). NIH3T3 and L929 cells, expressing CD300f ΔCT at levels equivalent to CD300f wild-type (WT) ( Supplementary Fig. 1 and Supplementary Fig. 3a ) engulfed significantly less AC than cells expressing CD300f WT, but more than the mock-transduced cells ( Fig. 3b,c and Supplementary Fig. 1 ), suggesting that CD300f provides both tethering and signalling cues. In addition, cells overexpressing WT protein were more efficient at the engulfment of PS liposome-coated beads than cells expressing ΔCT ( Fig. 3d,e ). 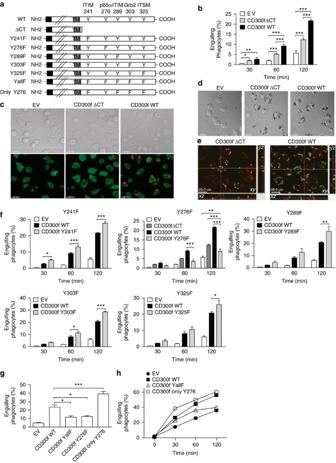Figure 3: The tyrosine-based motifs in CD300f cytoplasmic tail initiate signals that differentially regulate the phagocytosis of AC. (a) Schematic representation of CD300f and its mutants used in the study. The amino-acid number of tyrosine residues located within putative tyrosine-based signalling motifs is indicated at the top. For the visualisation purpose, the size of extracellular portion is reduced and drawn not to scale. (b) L929 cells transduced with the indicated constructs were mixed with TFL-4-labeled AC at a 1:3 ratio for the indicated times. Cells were then fixed and analysed by flow cytometry for the percentage of cells containing AC, as forFig. 2a. The graph shows means with s.e.m. (error bars) from three experiments; asterisks indicate statistical significance (*P<0.05, **P<0.01, ***P<0.001; two-way analysis of variance, ANOVA). (c) CFSE-labelled L929 cells, transduced with the indicated constructs, were mixed with pHrodo-labelled AC at a 1:15 ratio. After 2 h, the cells were analysed by confocal microscopy as forFig. 1a. The top row shows the DIC images; the bottom row shows the CFSE-labelled L929 cells (green) and the engulfed pHrodo-labelled AC (red). Scale bars, 20 μm. (d,e) L929 cells transduced with the indicated constructs were mixed with PS liposome-coated beads for 1 h. Cells were washed, fixed, permeabilized, stained by phalloidin and analysed by confocal microscopy. Representative single optical sections are shown in DIC images in (d). The images in (e) show the images in all three axes; F-actin is red, green indicates the auto-fluorescence of liposome-coated beads; scale bars, 20 μm. (f,g) L929 cells stably transduced with the indicated constructs were mixed with TFL-4-labeled AC at a 1:3 ratio for the indicated times. Cells were fixed and analysed by flow cytometry as inFig. 2a. The graphs show the mean values with s.e.m. (error bars) from three experiments; asterisks indicate statistical significance (*P<0.05, **P<0.01, ***P<0.001; two-way ANOVA in f, Student’st-test ing). (h) BMDM fromCd300f−/−mice transduced with the indicated constructs were mixed with pHrodo-labelled AC at a 1:3 ratio for the indicated times, suspended in basic buffer and analysed by flow cytometry as inFig. 1. The graph illustrates the representative of three experiments. Figure 3: The tyrosine-based motifs in CD300f cytoplasmic tail initiate signals that differentially regulate the phagocytosis of AC. ( a ) Schematic representation of CD300f and its mutants used in the study. The amino-acid number of tyrosine residues located within putative tyrosine-based signalling motifs is indicated at the top. For the visualisation purpose, the size of extracellular portion is reduced and drawn not to scale. ( b ) L929 cells transduced with the indicated constructs were mixed with TFL-4-labeled AC at a 1:3 ratio for the indicated times. Cells were then fixed and analysed by flow cytometry for the percentage of cells containing AC, as for Fig. 2a . The graph shows means with s.e.m. (error bars) from three experiments; asterisks indicate statistical significance (* P <0.05, ** P <0.01, *** P <0.001; two-way analysis of variance, ANOVA). ( c ) CFSE-labelled L929 cells, transduced with the indicated constructs, were mixed with pHrodo-labelled AC at a 1:15 ratio. After 2 h, the cells were analysed by confocal microscopy as for Fig. 1a . The top row shows the DIC images; the bottom row shows the CFSE-labelled L929 cells (green) and the engulfed pHrodo-labelled AC (red). Scale bars, 20 μm. ( d , e ) L929 cells transduced with the indicated constructs were mixed with PS liposome-coated beads for 1 h. Cells were washed, fixed, permeabilized, stained by phalloidin and analysed by confocal microscopy. Representative single optical sections are shown in DIC images in ( d ). The images in ( e ) show the images in all three axes; F-actin is red, green indicates the auto-fluorescence of liposome-coated beads; scale bars, 20 μm. ( f , g ) L929 cells stably transduced with the indicated constructs were mixed with TFL-4-labeled AC at a 1:3 ratio for the indicated times. Cells were fixed and analysed by flow cytometry as in Fig. 2a . The graphs show the mean values with s.e.m. (error bars) from three experiments; asterisks indicate statistical significance (* P <0.05, ** P <0.01, *** P <0.001; two-way ANOVA in f, Student’s t -test in g ). ( h ) BMDM from Cd300f − / − mice transduced with the indicated constructs were mixed with pHrodo-labelled AC at a 1:3 ratio for the indicated times, suspended in basic buffer and analysed by flow cytometry as in Fig. 1 . The graph illustrates the representative of three experiments. Full size image The cytoplasmic tail of CD300f possesses five putative tyrosine phosphorylation sites ( Fig. 3a ) residing in potential signalling motifs [28] . To investigate their role in phagocytosis, we created CD300f mutants with each tyrosine converted to phenylalanine ( Fig. 3a ) and stably expressed them to similar levels in L929 cells ( Supplementary Fig. 3a ). Relative to CD300f WT, expression of Y276F mutant markedly decreased the level of AC phagocytosis by ~60%, whereas expression of each of the other mutants slightly increased the phagocytic level by ~20% on average ( Fig. 3f ). We obtained similar results using cell clones with equivalent CD300f expression levels ( Supplementary Fig. 4 ). These data imply that the Y276-based motif recruits a protein(s) capable of initiating signals promoting phagocytosis, while the other tyrosine-based motifs bind proteins that initiate inhibitory signals. Additionally, we created L929 cells expressing equivalent levels of CD300f mutants that had all the tyrosines converted to phenylalanine (YallF), or all but Y276 (Only-Y276) ( Fig. 3a and Supplementary Fig. 3a ). Compared with CD300f WT cells, the cells expressing Only-Y276 mutant showed significantly increased phagocytosis (70%), whereas YallF or Y276F cell showed substantially decreased phagocytosis (~50%) ( Fig. 3g ). Furthermore, when overexpressed in J774 macrophages ( Supplementary Fig. 3b ), Only-Y276 mediated the most phagocytosis, indicating that the Y276-based motif also initiates positive signals in macrophages ( Supplementary Fig. 3c ). Next, we transduced BMDM from Cd300f −/− mice with CD300f WT or mutants ( Supplementary Fig. 3d ). The knock-in of CD300f WT or Only-Y276 resulted in enhanced AC phagocytosis ( Fig. 3h ), demonstrating that CD300f indeed functions in positive regulation of phagocytosis. The signalling-defective CD300f YallF showed more phagocytosis than the empty virus-transduced CD300f-deficient BMDM, in line with its tethering ability. Collectively, these data indicate that PS recognition by CD300f promotes AC phagocytosis due primarily to the positive signals emanating from Y276-based motif in the cytoplasmic tail. CD300f associates with p85α and SHP1 Since our results indicated that tyrosine-based motifs are important for CD300f function, we examined CD300f phosphorylation. CD300f tyrosine phosphorylation was markedly increased in response to AC stimulation ( Fig. 4a and uncropped gel image in Supplementary Fig. 5a ). Y276 exhibited prominent phosphorylation, Y303 phosphorylation was also readily detectable, while the other tyrosines showed only trace levels of phosphorylation ( Fig. 4a and uncropped gel image in Supplementary Fig. 5a ). The Y276-based motif is a putative-binding site for the PI3K subunit p85α ( Fig. 3a ); indeed, p85α weakly associated with CD300f WT in non-stimulated cells and the binding was enhanced sixfold following AC stimulation ( Fig. 4b and uncropped gel image in Supplementary Fig. 5b ). The CD300f Only-Y276 mutant had enhanced association with p85α compared with WT ( Fig. 4b and uncropped gel image in Supplementary Fig. 5b ), which agrees with the enhanced phagocytic activity of this mutant ( Fig. 3g ). CD300f YallF and Y276F mutants did not show any detectable binding of p85α ( Fig. 4b and uncropped gel image in Supplementary Fig. 5b ), indicating that phosphorylated Y276 is required for the interaction with PI3K. 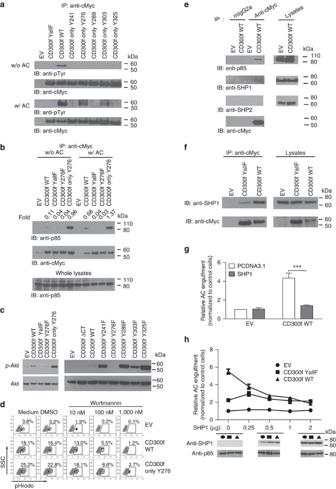Figure 4: CD300f associates with p85α subunit of PI3K and SHP1 to regulate the phagocytosis of AC. (a–c) L929 cells transduced with EV or cMyc-tagged CD300f constructs were incubated with (a–c) or without (a,b) AC at 4 °C for 10 min, then transferred to 37 °C for 15 min before lysis. Immunoprecipitation was performed with anti-cMyc Ab (a,b), and blotting with antibodies against phosphotyrosine (a), p85 (b) or cMyc (a,b) (loading control). The presence of PI3K subunit was verified by anti-p85 immunoblotting of whole lysates (b); anti-phospho-Akt or anti-Akt (loading control) blots were performed on whole lysates (c). (d) L929 cells transduced with the indicated constructs were preincubated with medium or DMSO (controls), or Wortmannin for 30 min at 37 °C, followed by 2 h incubation with pHrodo-labelled AC. The percentage of cells containing AC was determined as inFig. 1. (e) J774 cells transduced with EV or cMyc-tagged CD300f WT were treated with pervanadate for 15 min at 37 °C, lysed, immunoprecipitated with anti-cMyc or isotype control antibodies and then blotted with anti-p85, anti-SHP1, anti-SHP2 or anti-cMyc antibodies. Lysates blotted with anti-p85, anti-SHP1 or anti-SHP2 antibodies served as controls. (f) The indicated cMyc-tagged CD300f constructs were co-transfected with SHP1 into HeLa cells. Cells, treated with pervanadate, were lysed, immunoprecipitated with anti-cMyc Ab and blotted with anti-SHP1 or anti-cMyc antibodies. Cell lysates were blotted with anti-SHP1 or anti-cMyc for SHP1 or CD300f presence. (g) EV or CD300f WT was co-transfected with pCDNA3.1 or SHP1 into HeLa cells. Cells were incubated with pHrodo-labelled AC for 2 h, and phagocytosis efficiency was analysed as inFig. 1, and expressed as relative values normalized to EV- and pCDNA3.1-transfected control cells. The graph shows means with s.e.m. (error bars) from three experiments. Asterisks indicate statistical significance (***P<0.001, Student’st-test). (h) The indicated amounts of SHP1-encoding vector were co-transfected with EV or CD300f constructs into HeLa cells. The ability of cells to phagocytize pHrodo-labelled AC was analysed as in (g) and plotted versus SHP1 transfection level. The graph shows means with s.e.m. (error bars) from three experiments. The images below the graph show representative anti-SHP1 blots of lysates from cells transfected with 0, 0.5 or 2 μg of SHP1-encoding vector. Anti-p85 immunoblotting served as loading control. Figure 4: CD300f associates with p85α subunit of PI3K and SHP1 to regulate the phagocytosis of AC. ( a – c ) L929 cells transduced with EV or cMyc-tagged CD300f constructs were incubated with ( a – c ) or without ( a , b ) AC at 4 °C for 10 min, then transferred to 37 °C for 15 min before lysis. Immunoprecipitation was performed with anti-cMyc Ab ( a , b ), and blotting with antibodies against phosphotyrosine ( a ), p85 ( b ) or cMyc ( a , b ) (loading control). The presence of PI3K subunit was verified by anti-p85 immunoblotting of whole lysates ( b ); anti-phospho-Akt or anti-Akt (loading control) blots were performed on whole lysates ( c ). ( d ) L929 cells transduced with the indicated constructs were preincubated with medium or DMSO (controls), or Wortmannin for 30 min at 37 °C, followed by 2 h incubation with pHrodo-labelled AC. The percentage of cells containing AC was determined as in Fig. 1 . ( e ) J774 cells transduced with EV or cMyc-tagged CD300f WT were treated with pervanadate for 15 min at 37 °C, lysed, immunoprecipitated with anti-cMyc or isotype control antibodies and then blotted with anti-p85, anti-SHP1, anti-SHP2 or anti-cMyc antibodies. Lysates blotted with anti-p85, anti-SHP1 or anti-SHP2 antibodies served as controls. ( f ) The indicated cMyc-tagged CD300f constructs were co-transfected with SHP1 into HeLa cells. Cells, treated with pervanadate, were lysed, immunoprecipitated with anti-cMyc Ab and blotted with anti-SHP1 or anti-cMyc antibodies. Cell lysates were blotted with anti-SHP1 or anti-cMyc for SHP1 or CD300f presence. ( g ) EV or CD300f WT was co-transfected with pCDNA3.1 or SHP1 into HeLa cells. Cells were incubated with pHrodo-labelled AC for 2 h, and phagocytosis efficiency was analysed as in Fig. 1 , and expressed as relative values normalized to EV- and pCDNA3.1-transfected control cells. The graph shows means with s.e.m. (error bars) from three experiments. Asterisks indicate statistical significance (*** P <0.001, Student’s t -test). ( h ) The indicated amounts of SHP1-encoding vector were co-transfected with EV or CD300f constructs into HeLa cells. The ability of cells to phagocytize pHrodo-labelled AC was analysed as in ( g ) and plotted versus SHP1 transfection level. The graph shows means with s.e.m. (error bars) from three experiments. The images below the graph show representative anti-SHP1 blots of lysates from cells transfected with 0, 0.5 or 2 μg of SHP1-encoding vector. Anti-p85 immunoblotting served as loading control. Full size image Consistently, following AC stimulation, both CD300f WT- and Only-Y276-derived signals resulted in enhanced phosphorylation of Akt, a kinase downstream of PI3K activity ( Fig. 4c , Supplementary Fig. 2d and uncropped gel image in Supplementary Fig. 5c ). Akt phosphorylation was also elevated in cells expressing other CD300f mutants ( Fig. 4c and uncropped gel image in Supplementary Fig. 5c ) in line with the finding that these mutations enhanced AC phagocytosis ( Fig. 3f ). Wortmannin, a PI3K inhibitor, significantly inhibited CD300f-mediated AC phagocytosis ( Fig. 4d ), further confirming that CD300f recognition of AC results in activation of PI3K and enhanced phagocytosis. Although CD300f was able to mediate an activating signal for phagocytosis through Y276 phosphorylation, the phosphorylation of the other four Tyr residues residing in the ITIM (immunoreceptor tyrosine-based inhibitory motif) and switch motifs generated inhibitory signals ( Fig. 3a,f ). Indeed, we detected an association of CD300f with SHP1, but not SHP2 in J774 cells or HeLa cells ( Fig. 4e,f and uncropped gel image in Supplementary Fig. 6a,b ). Importantly, overexpression of SHP1 in HeLa cells decreased CD300f-mediated phagocytosis ( Fig. 4g ), and the inhibitory effects correlated positively with phosphatase expression levels ( Fig. 4h and uncropped gel image in Supplementary Fig. 6c ). CD300f signals actin rearrangements at the phagocytic cup After AC stimulation, the frequency of cells containing F-actin patches on the cell surface was twofold higher for cells expressing CD300f WT than cells expressing ΔCT ( Fig. 5a,b ). Similarly, L929 cells expressing CD300f Only-Y276 but not those expressing Y276F formed distinct F-actin clusters on the cell surface ( Fig. 5c , Supplementary Movie 1,2 ), suggesting that CD300f-mediated signalling affects actin cytoskeleton rearrangements. 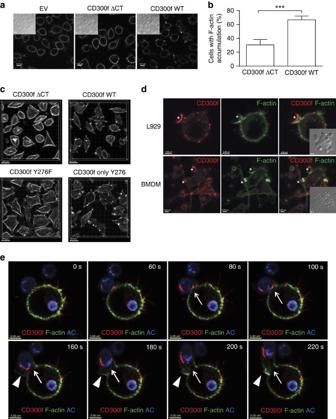Figure 5: CD300f clusters and F-actin assembly at the phagocytic cups. (a) L929 cells transduced with EV, CD300f ΔCT or CD300f WT were incubated with AC for 10 min at 4 °C, then transferred to 37 °C for 30 min. Cells were fixed, permeabilized and stained with Alexa Fluor568-conjugated phalloidin to visualize F-actin. The inserts show DIC images; scale bars, 10 μm. (b) Quantification of the percentage of phagocytes with F-actin patches on the cell surface, visualized as in (a). The data represent the means with s.e.m. (error bars) from the analysis of 100 cells from random fields of view (7 for CD300f ΔCT, 10 for CD300f WT). Asterisks indicate statistical significance (***P<0.001, Student’st-test). (c) L929 cells transduced with CD300f WT, CD300f ΔCT, CD300f Y276F or CD300f Only-Y276 were incubated with AC and stained with phalloidin as in (a). Multiple optical sections were acquired, and 3D reconstruction images were generated to visualize F-actin in the entire cells. Scale bars, 20 μm. (d) L929 and BMDM cells expressing cMyc-tagged CD300f WT were cultured in a glass bottom dishes and incubated with AC for 30 min at 37 °C. The cells were then fixed, washed and stained using anti-cMyc Ab, followed by Alexa Fluor 647-conjugated secondary antibody (red). F-actin was stained using phalloidin-Alexa Fluor 568 (green). Asterisks indicate the position of AC. The inserts show DIC images; scale bars, 5 μm. (e) L929 cells expressing CD300f Only-Y276-EGFP mutant and Life-Act-RFP were incubated with TFL-4-labeled AC for 10 min at 4 °C, then were transferred to a heated chamber (37 °C). The process of AC engulfment was recorded by time-lapse microscopy. The images show the location of CD300f Only-Y276 (red), F-actin (green) and AC (blue) at the indicated time points during the engulfment process. The time point when CD300f started to cluster at the contact site with the AC was assigned as time zero (0 s). Arrows indicate CD300f clusters with hypo-dense F-actin present at the invaginating part of phagocytic cup; arrowheads point to F-actin reassembling at the protruding part of phagocytic cup. Scale bars, 5 μm. Figure 5: CD300f clusters and F-actin assembly at the phagocytic cups. ( a ) L929 cells transduced with EV, CD300f ΔCT or CD300f WT were incubated with AC for 10 min at 4 °C, then transferred to 37 °C for 30 min. Cells were fixed, permeabilized and stained with Alexa Fluor568-conjugated phalloidin to visualize F-actin. The inserts show DIC images; scale bars, 10 μm. ( b ) Quantification of the percentage of phagocytes with F-actin patches on the cell surface, visualized as in ( a ). The data represent the means with s.e.m. (error bars) from the analysis of 100 cells from random fields of view (7 for CD300f ΔCT, 10 for CD300f WT). Asterisks indicate statistical significance (*** P <0.001, Student’s t -test). ( c ) L929 cells transduced with CD300f WT, CD300f ΔCT, CD300f Y276F or CD300f Only-Y276 were incubated with AC and stained with phalloidin as in ( a ). Multiple optical sections were acquired, and 3D reconstruction images were generated to visualize F-actin in the entire cells. Scale bars, 20 μm. ( d ) L929 and BMDM cells expressing cMyc-tagged CD300f WT were cultured in a glass bottom dishes and incubated with AC for 30 min at 37 °C. The cells were then fixed, washed and stained using anti-cMyc Ab, followed by Alexa Fluor 647-conjugated secondary antibody (red). F-actin was stained using phalloidin-Alexa Fluor 568 (green). Asterisks indicate the position of AC. The inserts show DIC images; scale bars, 5 μm. ( e ) L929 cells expressing CD300f Only-Y276-EGFP mutant and Life-Act-RFP were incubated with TFL-4-labeled AC for 10 min at 4 °C, then were transferred to a heated chamber (37 °C). The process of AC engulfment was recorded by time-lapse microscopy. The images show the location of CD300f Only-Y276 (red), F-actin (green) and AC (blue) at the indicated time points during the engulfment process. The time point when CD300f started to cluster at the contact site with the AC was assigned as time zero (0 s). Arrows indicate CD300f clusters with hypo-dense F-actin present at the invaginating part of phagocytic cup; arrowheads point to F-actin reassembling at the protruding part of phagocytic cup. Scale bars, 5 μm. Full size image To further explain the relationship between CD300f and F-actin accumulation, we examined their location during AC phagocytosis. The portion of the phagocytic cup contacting the AC is referred to as the invaginating part, and the cup’s outer-edge as the protruding part ( Supplementary Fig. 7a ). CD300f was seen to form clusters at the AC contact sites with L929 or BMDM, and was located in the invaginating part of formed phagocytic cups ( Figs 5d,e and 6 , Supplementary Movie 3 ). CD300f accumulation was dependent on ligand recognition, and independent of its signalling capacity, as CD300f ΔCT also clustered at the AC contact sites, whereas LAIR-1, a collagen-recognizing receptor, and CD300f D117A were not enriched ( Supplementary Fig. 7b,c and Fig. 6a ). Moreover, CD300f accumulation was independent and upstream of actin rearrangements, as latrunculin A treatment that completely blocked AC phagocytosis ( Supplementary Fig. 7d ) did not inhibit CD300f clustering ( Supplementary Fig. 7e and Supplementary Movie 4 ). Interestingly, accumulated F-actin was mainly located on the protruding part of the cup, whereas the invaginating part exhibited hypo-dense or little F-actin ( Figs 5d,e and 6b ). Furthermore, the initial CD300f clusters preceded the F-actin disassembly on the invaginating part, which was followed later by F-actin reassembly on the protruding part, implying again that CD300f ligation leads to the rearrangement of actin cytoskeleton ( Fig. 5e ). 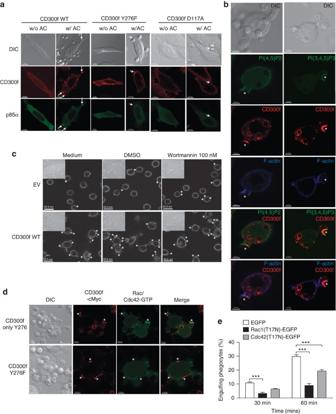Figure 6: CD300f-mediated PI3K-Rac/Cdc42 activation at the phagocytic cups. (a) cMyc-tagged CD300f WT, Y276F or D117A were co-transfected with p85α-YFP into HeLa cells. The cells were placed in glass bottom dishes without (w/o AC) or with AC (w/AC) at 4 °C for 10 min, and then transferred to 37 °C for 15 min. Cells were fixed, permeabilized, blocked and stained by anti-cMyc Ab, followed by Alexa Fluor 647-conjugated secondary antibody to visualize CD300f (red); p85 was visualized by YFP fluorescence (green). The arrows indicate clusters of CD300f and/or p85α at AC contact sites; scale bars, 10 μm. (b) L929 cells expressing cMyc-tagged CD300f Only-Y276 were transduced with PLCδ1-PH-YFP or Btk-PH-YFP probes, to visualize PI(4,5)P2 and PI(3,4,5)P3, respectively (green). Cells were incubated with AC at 37 °C for 30 min, and then immunostained for CD300f as in (a) (red). F-actin was stained with phalloidin-AlexaFluor 568 (blue). Scale bars, 5 μm. (c) L929 cells transduced with EV or CD300f were preincubated with medium or DMSO (controls), or 100 nM Wortmannin for 30 min at 37 °C. AC were mixed with L929 cells for 10 min at 4 °C, and then transferred for 30 min to 37 °C (in the presence of DMSO or Wortmannin). Cells were fixed, permeabilized and stained with Alexa Fluor568-conjugated phalloidin to visualize F-actin. The inserts show DIC images; asterisks indicate the AC position. Scale bars, 20 μm. (d) L929 cells expressing cMyc-tagged CD300f Y276F or Only-Y276 were transfected with an activated Rac/Cdc42 probe, PBD-EYFP. The cells were then incubated with AC at 4 °C for 10 min, and transferred to 37 °C for 15 min. Cells were fixed, washed and CD300f (red) and active Rac1/Cdc42 (green) were visualized as in (b). Asterisks indicate the AC position; scale bars, 5 μm. (e) NIH3T3 cells expressing CD300f WT were transfected with a dominant-negative form of Rac1 (Rac1(T17N)-EGFP) or Cdc42 (Cdc42(T17N)-EGFP), or EGFP control. The cells were mixed with TFL-4-labeled AC at a 1:3 ratio for the indicated times, and analysed by flow cytometry. The graph illustrates the percentage of TFL-4+cells from the GFP-positive population, representing the transfected NIH3T3 cells that engulfed AC. The graph shows the means with s.e.m. (error bars) from three experiments. Asterisks indicate statistical significance (***P<0.001, two-way ANOVA). Figure 6: CD300f-mediated PI3K-Rac/Cdc42 activation at the phagocytic cups. ( a ) cMyc-tagged CD300f WT, Y276F or D117A were co-transfected with p85α-YFP into HeLa cells. The cells were placed in glass bottom dishes without (w/o AC) or with AC (w/AC) at 4 °C for 10 min, and then transferred to 37 °C for 15 min. Cells were fixed, permeabilized, blocked and stained by anti-cMyc Ab, followed by Alexa Fluor 647-conjugated secondary antibody to visualize CD300f (red); p85 was visualized by YFP fluorescence (green). The arrows indicate clusters of CD300f and/or p85α at AC contact sites; scale bars, 10 μm. ( b ) L929 cells expressing cMyc-tagged CD300f Only-Y276 were transduced with PLCδ1-PH-YFP or Btk-PH-YFP probes, to visualize PI(4,5)P2 and PI(3,4,5)P3, respectively (green). Cells were incubated with AC at 37 °C for 30 min, and then immunostained for CD300f as in ( a ) (red). F-actin was stained with phalloidin-AlexaFluor 568 (blue). Scale bars, 5 μm. ( c ) L929 cells transduced with EV or CD300f were preincubated with medium or DMSO (controls), or 100 nM Wortmannin for 30 min at 37 °C. AC were mixed with L929 cells for 10 min at 4 °C, and then transferred for 30 min to 37 °C (in the presence of DMSO or Wortmannin). Cells were fixed, permeabilized and stained with Alexa Fluor568-conjugated phalloidin to visualize F-actin. The inserts show DIC images; asterisks indicate the AC position. Scale bars, 20 μm. ( d ) L929 cells expressing cMyc-tagged CD300f Y276F or Only-Y276 were transfected with an activated Rac/Cdc42 probe, PBD-EYFP. The cells were then incubated with AC at 4 °C for 10 min, and transferred to 37 °C for 15 min. Cells were fixed, washed and CD300f (red) and active Rac1/Cdc42 (green) were visualized as in ( b ). Asterisks indicate the AC position; scale bars, 5 μm. ( e ) NIH3T3 cells expressing CD300f WT were transfected with a dominant-negative form of Rac1 (Rac1(T17N)-EGFP) or Cdc42 (Cdc42(T17N)-EGFP), or EGFP control. The cells were mixed with TFL-4-labeled AC at a 1:3 ratio for the indicated times, and analysed by flow cytometry. The graph illustrates the percentage of TFL-4 + cells from the GFP-positive population, representing the transfected NIH3T3 cells that engulfed AC. The graph shows the means with s.e.m. (error bars) from three experiments. Asterisks indicate statistical significance (*** P <0.001, two-way ANOVA). Full size image To address how CD300f could signal actin rearrangements, we first visualized the association between CD300f and PI3K following AC stimulation. p85α formed clusters colocalizing with CD300f at the AC contact sites ( Fig. 6a ); CD300f Y276F also accumulated at the AC contact site, but did not recruit p85α, indicating that CD300f is responsible for the recruitment of PI3K to the phagocytic cups. PI3K catalyses the conversion of phosphatidylinositol-4,5-bisphosphate, PI(4,5)P2, to phosphatidylinositol-3,4,5-triphosphate, PI(3,4,5)P3 (ref. 12 ). Thus, we analysed the location of PI(4,5)P2 and PI(3,4,5)P3 during phagocytosis, using the probes PLCδ1-PH and Btk-PH [37] , respectively, and the CD300f Only-Y276 mutant that had the most robust interaction with PI3K. Following the binding of AC, PI(3,4,5)P3 was enriched at the invaginating part of the cups where CD300f clusters were present, whereas PI(4,5)P2 and F-actin were absent from these sites ( Fig. 6b , Supplementary Movie 5,6 ). Considering the roles of PI(4,5)P2 and PI(3,4,5)P3 in actin rearrangements [12] , [38] , [39] , this suggests that CD300f-mediated PI3K activation regulates the rearrangement of actin at the phagocytic cups. Indeed, Wortmannin treatment inhibited the formation of F-actin patches mediated by CD300f ( Fig. 6c ). The small GTPase Rac/Cdc42 functions downstream of PI3K to regulate actin rearrangement [40] , [41] . PBD-EYFP, a probe for the active form of Rac/Cdc42 (ref. 42 ), revealed that activated Rac/Cdc42 was recruited to the phagocytic cups and colocalized with CD300f WT but not with Y276F ( Fig. 6d ). Overexpression of Rac1(T17N) or Cdc42(T17N) dominant-negative mutants in NIH3T3 cells efficiently inhibited CD300f-mediated AC phagocytosis ( Fig. 6e ). These data indicate that accumulated CD300f on the phagocytic cups activates the PI3K-Rac/Cdc42 pathway for actin rearrangement, thus enhancing AC phagocytosis. CD300f deficiency accelerates systemic autoimmune disease Defects in AC clearance are associated with the spontaneous or accelerated autoimmune disease development in mice [16] , [43] , [44] , [45] , [46] , [47] , [48] , [49] . We therefore investigated whether CD300f deficiency plays a role in the development of autoimmunity. We found no overt signs of autoimmune disease in CD300f-deficient mice. We asked then whether CD300f deficiency could accelerate the development of autoimmune disease in C57BL/6 Fcgr2b −/− mice that are prone to develop fatal glomerulonephritis [50] . We created Cd300f −/− Fcgr2b −/− mice and found they exhibited both accelerated and increased overall mortality relative to the parental strains ( Fig. 7a ). Splenomegaly, observed in both Fcgr2b −/− and Cd300f −/− Fcgr2b −/− mice was more severe at 8 months in Cd300f −/− Fcgr2b −/− mice than in mice deficient in FcγRIIB ( Fig. 7b ). Cd300f −/− Fcgr2b −/− mice showed significant elevations in both spleen weight and total cell numbers ( Fig. 7c,d ). Levels of anti-dsDNA antibodies were also significantly increased in sera from Cd300f −/− Fcgr2b −/− mice ( Fig. 7e ), and HEp-2 cells showed more intense anti-nuclear antibody (ANA) staining with sera from Cd300f −/− Fcgr2b −/− mice ( Fig. 7f,g ). In addition, the glomerular deposition of immunoglobulin G (IgG) and complement C3 was more pronounced in kidneys of Cd300f −/− Fcgr2b −/− mice ( Fig. 7h ), indicative of enhanced tissue pathology. Indeed, the hematoxylin and eosin-stained tissue sections from the kidney, liver, lung and spleen of Cd300f −/− Fcgr2b −/− mice revealed systemic vasculitis characterized by inflammatory cell infiltration, which was absent or rarely seen in other mouse strains tissues ( Fig. 7i ). Notably, Cd300f −/− Fcgr2b −/− mice developed significant glomerulonephritis associated with the widespread presence of tubular casts ( Fig. 7i ). Analyses of Cd300f −/− Fcgr2b −/− mouse spleen sections also revealed loss of normal follicular architecture, reduced red pulp and prominent areas of plasmacytosis ( Fig. 7i ). Thus, our results indicate that CD300f deficiency can serve to accelerate the development of autoimmunity. 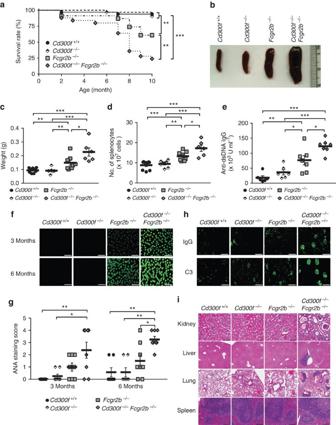Figure 7: CD300f deficiency accelerates systemic autoimmune disease inFcgr2b−/−mice. (a) Survival ofCd300f+/+(n=33),Cd300f−/−(n=32),Fcgr2b−/−(n=23) andCd300f−/−Fcgr2b−/−(n=25) mice was determined according to the Kaplan–Meier methodology. Asterisks indicate statistical significance (**P<0.01, ***P<0.005, the Mantel–Cox test). (b) Photograph of representative spleens isolated from 8 months oldCd300f+/+,Cd300f−/−,Fcgr2b−/−andCd300f−/−Fcgr2b−/−mice. (c,d) Spleen weight (c) and the total number of splenocytes (d) from 8 months oldCd300+/+,Cd300f−/−,Fcgr2b−/−andCd300f−/−Fcgr2b−/−mice. Each symbol represents a mouse. Data represent the means±s.e.m. (error bars). Asterisks indicate statistical significance (*P<0.05, **P<0.01, ***P<0.005, Student’st-test). (e) The serum levels of anti-dsDNA IgG in 6-month-old mice were measured by enzyme-linked immunosorbent assay (ELISA). Each symbol represents a mouse. Data represent the means±s.e.m. (error bars). Asterisks indicate statistical significance (*P<0.05, **P<0.01, ***P<0.005, Student’st-test). (f) Representative ANA stains of fixed HEp-2 cells with sera (1:200 dilution) from 3 to 6 months oldCd300f+/+,Cd300f−/−,Fcgr2b−/−andCd300−/−Fcgr2b−/−mice. Scale bars, 100 μm. (g) The summary of ANA intensity score quantification, determined as described in Methods. Each symbol represents a mouse. Data represent the means±s.e.m. (error bars). Asterisks indicate statistical significance (*P<0.05, **P<0.01, Student’st-test). (h) Kidney sections from 9 months oldCd300f+/+,Cd300f−/−,Fcgr2b−/−andCd300f−/−Fcgr2b−/−mice were stained with FITC-conjugated goat anti-mouse IgG or FITC-conjugated goat F(ab′)2anti-mouse C3 Ab, to visualize the kidney deposition of immunoglobulin and complement component 3, respectively. Scale bars, 100 μm. (i) Formalin-fixed paraffin-embedded tissue sections of the kidney, liver, lung and spleen from 9 months oldCd300f+/+,Cd300f−/−,Fcgr2b−/−andCd300f−/−Fcgr2b−/−mice were analysed using hematoxylin and eosin (H&E) staining. Data are representative of two to three mice per each genotype mice. Scale bars, 100 μm. Figure 7: CD300f deficiency accelerates systemic autoimmune disease in Fcgr2b −/− mice. ( a ) Survival of Cd300f +/+ ( n =33), Cd300f −/− ( n =32), Fcgr2b −/− ( n =23) and Cd300f −/− Fcgr2b −/− ( n =25) mice was determined according to the Kaplan–Meier methodology. Asterisks indicate statistical significance (** P <0.01, *** P <0.005, the Mantel–Cox test). ( b ) Photograph of representative spleens isolated from 8 months old Cd300f +/+ , Cd300f −/− , Fcgr2b −/− and Cd300f −/− Fcgr2b −/− mice. ( c , d ) Spleen weight ( c ) and the total number of splenocytes ( d ) from 8 months old Cd300 +/+ , Cd300f −/− , Fcgr2b −/− and Cd300f −/− Fcgr2b −/− mice. Each symbol represents a mouse. Data represent the means±s.e.m. (error bars). Asterisks indicate statistical significance (* P <0.05, ** P <0.01, *** P <0.005, Student’s t -test). ( e ) The serum levels of anti-dsDNA IgG in 6-month-old mice were measured by enzyme-linked immunosorbent assay (ELISA). Each symbol represents a mouse. Data represent the means±s.e.m. (error bars). Asterisks indicate statistical significance (* P <0.05, ** P <0.01, *** P <0.005, Student’s t -test). ( f ) Representative ANA stains of fixed HEp-2 cells with sera (1:200 dilution) from 3 to 6 months old Cd300f +/+ , Cd300f −/− , Fcgr2b −/− and Cd300 −/− Fcgr2b −/− mice. Scale bars, 100 μm. ( g ) The summary of ANA intensity score quantification, determined as described in Methods. Each symbol represents a mouse. Data represent the means±s.e.m. (error bars). Asterisks indicate statistical significance (* P <0.05, ** P <0.01, Student’s t -test). ( h ) Kidney sections from 9 months old Cd300f +/+ , Cd300f −/− , Fcgr2b −/− and Cd300f −/− Fcgr2b −/− mice were stained with FITC-conjugated goat anti-mouse IgG or FITC-conjugated goat F(ab′) 2 anti-mouse C3 Ab, to visualize the kidney deposition of immunoglobulin and complement component 3, respectively. Scale bars, 100 μm. ( i ) Formalin-fixed paraffin-embedded tissue sections of the kidney, liver, lung and spleen from 9 months old Cd300f +/+ , Cd300f −/− , Fcgr2b −/− and Cd300f −/− Fcgr2b −/− mice were analysed using hematoxylin and eosin (H&E) staining. Data are representative of two to three mice per each genotype mice. Scale bars, 100 μm. Full size image Here we identify and characterize the function of CD300f. We show that CD300f-mediated phagocytosis of AC occurs in a PS-dependent manner, as annexin V, MFG-E8 or PS-containing liposomes block CD300f-mediated phagocytosis. Additionally, cells expressing CD300f phagocytize beads coated with PS-liposomes. It is important to note that a membrane environment is most likely critical for CD300f binding to PS, as it has been difficult to detect CD300f binding to PS, which is extraneous of liposomes [19] , [34] , [35] . Even though PG can also be recognized by CD300f, the facts that PG is not commonly found in eukaryotic plasma membranes and that MFG-E8, which is PS specific, completely blocks CD300f-mediated phagocytosis rule out a significant role for PG in CD300f-mediated phagocytosis of ACs. CD300f was recently reported to bind ceramide. However, we found that liposomes containing ceramide failed to block CD300f-mediated phagocytosis, indicating that, in contrast to PS, ceramide does not play an important role in the function of CD300f as a molecule mediating recognition and engulfment of AC. Impaired AC clearance is often associated with the development of autoimmunity, as is seen in mice deficient in expression of several PS-recognition proteins [44] , [46] , [48] , [49] . Surprisingly, C57BL/6 mice deficient in CD300f are relatively healthy, which may be due to their genetic background and the redundancy in PS-recognition receptors. For instance, MFG-E8-deficient mice produce autoantibodies on a mixed 129/B6 background but not on a C57BL/6 genetic background [48] , [49] . In addition, mice deficient in TIM4 develop little or no autoantibodies on C57BL/6 background, unless the mice are also deficient in MFG-E8 (refs 46 , 49 ). Similarly, mice deficient in both FcγRIIB, which predisposes to systemic lupus erythematosus [50] and CD300f exhibit an accelerated and more lethal course of autoimmune disease, associated with splenomegaly, autoantibody production and tissue pathology. Thus, the impaired clearance of AC associated with CD300f deficiency exacerbates the development of autoimmunity. CD300f expression clearly promotes AC phagocytosis by primary macrophages and cell lines, in a manner that is largely dependent on the capacity of CD300f to signal. We show that AC recognition strongly enhances the phosphorylation of CD300f tyrosine, predominantly on Y276, which leads to p85α recruitment to CD300f. This is followed by activation of PI3K, as demonstrated by the production of PI(3,4,5)P3 and Akt phosphorylation. The phosphorylation of the other four tyrosines leads to inhibition of phagocytosis by inhibiting PI3K activation, as evidenced by changes in Akt phosphorylation. A mutation of any one of the four tyrosines resulted in the increased AC phagocytosis, indicating that those tyrosine-based motifs are indeed involved in the initiation of an inhibitory signal. Most likely, SHP1 is the phosphatase involved in the inhibitory signalling, as it associates with CD300f in J774 and HeLa cells, and SHP1 overexpression decreases CD300f-mediated AC phagocytosis in a dose-dependent manner. In agreement, SHP1 has been shown to be recruited to Fc receptor-mediated phagosomes and negatively regulate phagocytosis [51] , [52] . The maximal association between CD300f and SHP1 has been reported to require several tyrosines (Y241, Y289 and Y325) [32] . Exactly how the multiple tyrosines cooperatively associate with SHP1 for the regulation of phagocytosis needs further study. Intriguingly, mouse CD300f has been shown to serve as an activating or inhibitory receptor [30] , [31] , [32] , [53] . Our data indicate that CD300f might function differently depending on the signalling capacity available within a cell type. In fibroblast cells, expression of CD300f WT generates positive signals resulting from phosphorylation of Y276 that dominate over negative signals. In J774 macrophages, however, the inhibitory cues appear to override the positive signal, as cells expressing CD300f WT or Y276F mutant showed reduced phagocytic activity compared with cells expressing signalling-deficient forms. A possible explanation could be that SHP1 is expressed at much higher levels in J774 cells than in L929 cells, which may lead to its more efficient recruitment by CD300f resulting in reduced PI3K activation. Alternatively, the inositol 5-phosphatase, SHIP1, expressed in J774 but not in L929 cells, could hydrolyse PI(3,4,5)P3 resulting in deactivation of PI3K. In this regard, SHIP1 was reported to be recruited to phagocytic cups and regulate phagocytosis of IgG-opsonized particles [37] . Even though we and others did not detect an association of SHIP1 with CD300f [30] , [32] , the phosphatase might be recruited to phagocytic cups by other, unknown receptors, and thus indirectly decrease the CD300f-initiated activation of PI3K in macrophage cells. Likewise, the recruitment of SHP1 by CD300f could down modulate positive signals for phagocytosis generated by other receptors. Thus, the availability of phosphatases could affect the functions played by CD300f in a particular cell type. PI3K kinase activity appears to be essential for phagocytosis, as PI3K inhibitors impair target engulfment for both Fc receptor- and PS-recognition receptor-mediated phagocytosis [8] , [54] . Local activation of PI3K is required to induce actin reorganization and subsequent uptake of IgG-opsonized targets [20] , [55] , presumably related to the PI3K requirement for pseudopodia extension [56] and generation of contractile force on phagosomes by the recruitment of myosin X [57] . In this study, we present the details about CD300f’s function in AC engulfment, highlighting the involvement of PI3K and actin rearrangements. We propose that CD300f accumulates at AC contact sites that will evolve into the invaginating part of phagocytic cups and where following phosphorylation in response to PS recognition, it recruits p85α and activates PI3K ( Fig. 8 ). This, in turn, results in PI3K phosphorylating PI(4,5)P2 to PI(3,4,5)P3. As PI(4,5)P2 associates with gelsolin, profilin and other proteins regulating actin cytoskeleton [8] , [38] , [39] , the absence of PI(4,5)P2 could lead to the clearance of cortical F-actin from the invaginating part of the cup during CD300f-mediated phagocytosis. This would eliminate a possible physical barrier created by the actin meshwork and decrease the membrane rigidity, thereby allowing for easier membrane deformation and AC internalization [8] . At the same time, the increase in PI(3,4,5)P3 levels would serve to activate the small GTPase Rac/Cdc42 pathway to promote F-actin assembly along the protruding part of the phagocytic cups for membrane extension, required for phagocytic cup closure ( Fig. 8 ). The fact that latrunculin treatment blocks CD300f-mediated protrusion extension and phagosome sealing without interruption of membrane cup formation supports the notion that F-actin is unnecessary for the initial membrane cup formation [58] , but is required for further cup extension and phagosome sealing. 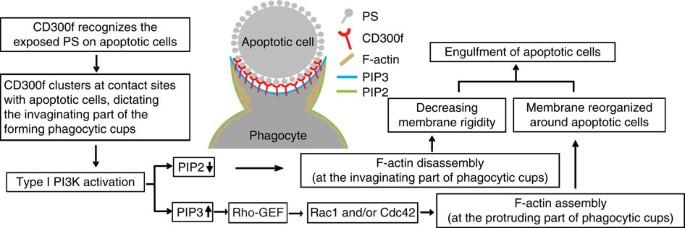Figure 8: Proposed model for CD300f-mediated phagocytosis of AC. During the encounter of a phagocyte with an AC, CD300f recognizes and binds PS exposed on the surface of AC, and accumulates at the nascent phagocytic cup sites, dictating the invaginating part. This leads to phosphorylation of CD300f, predominantly on the tyrosine 276, and recruitment of the regulatory subunit of PI3K, p85α. In turn, the activated PI3K catalyses the conversion of PI(4,5)P2 (PIP2) to PI(3,4,5)P3 (PIP3). The PI3K-mediated decrease in the PIP2 levels at the invaginating part of phagocytic cups leads to a local cortical actin depolymerisation and/or generation of actin meshwork hypo-density, and thus decreasing membrane rigidity and removing a physical barrier that could impair the engulfment of apoptotic cell. At the same time, the PI3K-induced increase of PIP3 levels promotes activation of Rac1/Cdc42 likely via the Rho-GEFs (guanine nucleotide exchange factors), leading to the stimulation of actin polymerization along the protruding part of the phagocytic cups. This drives the membrane reorganization around AC and results in phagocytic cup closure and AC engulfment. Thus, the CD300f-mediated signal promotes the phagocytosis of AC through changes in the levels of phosphoinositol second messenger system that leads to activation of proteins involved in actin cytoskeleton rearrangements and, consequently, local changes in actin organization and membrane dynamics at the phagocytic cups. Figure 8: Proposed model for CD300f-mediated phagocytosis of AC. During the encounter of a phagocyte with an AC, CD300f recognizes and binds PS exposed on the surface of AC, and accumulates at the nascent phagocytic cup sites, dictating the invaginating part. This leads to phosphorylation of CD300f, predominantly on the tyrosine 276, and recruitment of the regulatory subunit of PI3K, p85α. In turn, the activated PI3K catalyses the conversion of PI(4,5)P2 (PIP2) to PI(3,4,5)P3 (PIP3). The PI3K-mediated decrease in the PIP2 levels at the invaginating part of phagocytic cups leads to a local cortical actin depolymerisation and/or generation of actin meshwork hypo-density, and thus decreasing membrane rigidity and removing a physical barrier that could impair the engulfment of apoptotic cell. At the same time, the PI3K-induced increase of PIP3 levels promotes activation of Rac1/Cdc42 likely via the Rho-GEFs (guanine nucleotide exchange factors), leading to the stimulation of actin polymerization along the protruding part of the phagocytic cups. This drives the membrane reorganization around AC and results in phagocytic cup closure and AC engulfment. Thus, the CD300f-mediated signal promotes the phagocytosis of AC through changes in the levels of phosphoinositol second messenger system that leads to activation of proteins involved in actin cytoskeleton rearrangements and, consequently, local changes in actin organization and membrane dynamics at the phagocytic cups. Full size image In summary, our report demonstrates that CD300f recognizes PS exposed on the AC surface, and transduces signals for PI3K activation and F-actin remodelling, thereby promoting AC phagocytosis. Consequently, a deficiency in CD300f leads to impaired AC clearance and exacerbates the development of autoimmune disease. Animals The Cd300f − / − C57BL/6 strain was generated by OZgene and the Fcgr2b −/− C57BL/6 mice were kindly supplied by Dr Silvia Bolland (National Institute of Allergy and Infectious Diseases, MD, USA). Mice were crossed to create the Cd300f − / − Fcgr2b − / − double knockout mice. All animals were bred and housed in a pathogen-free environment in the NIAID animal facility with experimental protocols (LIG5E) approved by the NIAID Animal Care and Use Committee. Except the mortality analysis with both male and female mice, the characterization of autoimmune disease was performed on female mice at the ages indicated in the appropriate figure legends. For the in vivo or in vitro phagocytosis by primary macrophages, 8–10-week-old female mice were used. Cells and antibodies L929, NIH3T3, HEK293T and J774 cells were cultured in DMEM medium with 10% fetal bovine serum (FBS). Bone marrow cells were isolated from femurs and tibias of wt or Cd300f − / − mice. Differentiation of BMDM was induced by culturing bone marrow cells in RPMI 1640 medium supplemented with 10% FBS and 20% L929-conditioned medium (source of macrophage colony-stimulating factor) for 7 days with one renewal of the culture medium. Alveolar and peritoneal cells were harvested from wt or Cd300f − / − mice by alveolar or peritoneal lavage with cold, sterile phosphate-buffered saline (PBS) and cultured in RPMI 1640 medium with 10% FBS. Anti-mouse CD300f Ab and isotype control goat IgG were from R&D; the antibodies were labelled with Alexa Fluor 488 using Alexa Fluor-488 Monoclonal Antibody Labelling Kit (Invitrogen), according to the manufacturer’s instructions. Anti-SHP1 antibody was from Abcam. Anti-p85 and anti-phosphotyrosine (4G10) antibodies were from Millipore. Anti-cMyc (9B11), -SHP2 (D50F2), -Akt and -phospho-Akt (D9E) antibodies were from Cell Signaling. Horseradish peroxidase (HRP)-conjugated anti-cMyc Ab (9E10) and HRP-conjugated secondary antibodies (donkey anti-goat and goat anti-mouse) were from Santa Cruz Biotechnology. Anti-mouse CD16/CD32 (93), FITC-conjugated anti-mouse CD11b (M1/70) and APC-conjugated anti-mouse F4/80 (BM8) antibodies were from eBioscience. FITC-conjugated anti-human IgG Fc-gamma fragment-specific Ab was from Jackson ImmunoResearch Laboratories Inc. DNA reagents Full-length and extracellular domain CD300f complementary DNA (cDNA) constructs were described previously [19] . The DNA sequence of the primers used for plasmid constructs is given in the Supplementary Table 1 . For CD300f lentiviral expression constructs, the PCR product was cloned into pCDH-EF1-T2A-puro (pCDH) vector (System Biosciences), using BamH1 and NotI sites; a cMyc tag was added at the C terminus of CD300f constructs, unless stated otherwise. Tyrosine to phenylalanine substitution mutations in the cytoplasmic tail, or aspartic acid to alanine substitution in the extracellular domain of CD300f were generated using mutagenic oligonucleotides and the QuickChange Site-directed Mutagenesis Kit (Stratagene), according to the manufacturer’s instructions. To generate the CD300f YallF mutant, individual tyrosine mutations were introduced sequentially, using cDNA of one mutant as a template for the next step of mutagenesis. CD300f Only-Y276, Only-Y241, Only-Y289, Only-Y303 or Only-Y325 mutants were made using CD300f YallF as the template, and changing phenylalanine back to tyrosine. The CD300f ΔCT mutant, lacking the entire cytoplasmic tail, was generated by the introduction of a stop codon right after the region encoding the transmembrane domain of CD300f. To generate enhanced green fluorescent protein (EGFP)-tagged CD300f, EGFP cDNA was added at the 3′ terminus of CD300f WT or CD300f mutant cDNA in pCDH vector. To create retrovirus constructs, cDNA of CD300f WT or CD300f mutants were cloned into pMX-puro vector, which was kindly supplied by Dr Shigekazu Nagata (Kyoto University, Kyoto, Japan). The LAIR-1-EGFP plasmid and EGFP-tagged dominant-negative form of Rac1(T17N) were described previously [59] , [60] . The dominant-negative form of Cdc42 (T17N) was generated using QuickChange Site-directed Mutagenesis Kit (Stratagene) with the Cdc42 plasmid as the template kindly supplied by Dr Debbie C. Thurmond (Indiana University School of Medicine, Indianapolis, IN, USA) and sub-cloned into pEGFP-N1 plasmid (Clontech). Human p85-YFP, PLCδ1-PH-YFP and Btk-PH-YFP expression plasmids were kindly supplied by Dr Joel A. Swanson (University of Michigan Medical School, MI, USA). PBD-EYFP plasmid was kindly supplied by Dr Klaus Hahn (University of North Carolina, Chapel Hill, NC, USA). Life-Act-RFP cDNA was from Ibidi GmbH. PLCδ1-PH-YFP, Btk-PH-YFP, and Life-Act-RFP were sub-cloned into the pCDH-puro vector, to generate the lentiviral expression constructs. Cell transfection and infection L929 or NIH3T3 cells were transfected with xTreme Fugene HD (Roche Diagnostics); HeLa and HEK293T cells were transfected using Lipofectamin 2000 (Invitrogen). Lentivirus particles were generated by co-transfection of HEK293T cells with pCDH-puro expression vectors encoding WT or mutated CD300f, and psPAX2 and pMD2G helper plasmids. Infections of L929, NIH3T3 and J774 cells were carried out by incubating the cells with lentiviruses for 24 h at 37 °C, in the presence of 8 μg ml −1 protamine sulphate (Sigma). Selection with puromycin (20 μg ml −1 for L929 or NIH3T3 cells; 6 μg ml −1 for J774 cells) was started 48 h after infection. For transformation of primary macrophages, the BMDM were seeded at 1 × 10 5 cells per ml in complete RPMI 1640 medium with 100 ng ml −1 macrophage colony-stimulating factor (eBioscience), and incubated with the retroviruses for 8 h at 37 °C in the presence of 6 μg ml −1 protamine sulphate. After infection, the cells were cultured in complete RPMI 1640 with 20% L929-conditioning medium for 36 h, followed by selection with 6 μg ml −1 puromycin (Sigma). Chimeric proteins 293T cells were transfected with pcDNA3.1 plasmids encoding CD300f/Fc, CD300f D117A/Fc and LAIR-1 R65K/Fc constructs using Lipofectamin (Invitrogen). Forty-eight hours after transfection, the culture supernatant, containing the chimeric proteins, was harvested and the Fc-fusion proteins were purified using protein A-Sepharose Fast Flow columns (Amersham Biosciences). On the basis of CD300f and annexin V sequence comparison, aspartic acid at position 117 of CD300f is predicted to be important for calcium, and consequently, PS binding. LAIR-1 R65K with markedly reduced avidity for the ligand collagens [60] was used as the negative control. Phospholipid-containing liposomes and liposome-coated beads Synthetic 1,2-dioleoyl-sn-glycero-3-phosphocholine (DOPC), 1,2-dioleoyl- sn- glycero-3-phospho- L -serine (DOPS), 1-palmitoyl-2-oleoyl- sn -glycero-3-phosphocholine (POPC), 1-palmitoyl-2-oleoyl- sn -glycero-3-phospho- L -serine (POPS), 1-palmitoyl-2-oleoyl- sn -glycero-3-phosphoethanolamine (POPE), 1-palmitoyl-2-oleoyl- sn -glycero-3-phospho-(1′- rac -glycerol) (POPG) and ceramide were from Avanti Polar Lipids. N-(biotinoyl)-1, 2-dihexadecanoyl-sn-glycero-3-phosphoethanolamine, triethylammonium (biotin-labelled DHPE) was from Invitrogen. Liposomes were prepared by completely evaporating the chloroform from the desired phospholipid mixture with argon gas. Large multilamellar vesicles were formed by swirling in degassed PBS (pH 7.4). Unilamellar vesicles were prepared by extrusion through filters with 100 nm pore size, using Avanti Mini-Extruder (Avanti Polar Lipids). Liposome composition was 80% DOPC and 20% of POPC, POPS, POPE, POPG or ceramide. For the liposomes used to coat the beads, the lipid composition was 99% DOPC: 1% biotin-labelled DHPE for PC liposome and 49% DOPC: 50% DOPS: 1% biotin-labelled DHPE for PS liposome. M-280 streptavidin-coated Dynabeads (Invitrogen) were first preincubated in PBS with 1% bovine serum albumin (BSA) (Sigma) at 37 °C for 2 h, then mixed with liposomes for 2 h at 37 °C in degassed PBS with 1% BSA, and followed by two washing steps and resuspension in the same buffer. The presence of PS on the beads was confirmed by staining with Annexin V-APC (eBioscience) and flow cytometry analysis. Liposomes and liposome-coated beads were stored in argon gas to prevented lipid oxidization. Phagocytosis assay Apoptotic thymocytes were generated by incubating the cells at 37 °C for 6 h with 10 μM dexamethasone (Sigma), at which time at least 80% of the cells were Annexin V positive. The ACs were labelled with TFL-4 (OncoImmunin) or pHrodo (Invitrogen), and added to the phagocytes at a 3:1, 5:1 or 15:1 ratio, as indicated in the text. After incubation, the phagocytes were washed, treated with trypsin/EDTA (L929 and NIH3T3 cells; Sigma) or accutase (J774 cells and primary macrophages; Innovative Cell Technologies Inc), fixed and analysed by flow cytometry or visualized by LSM710 laser scanning confocal microscopy (Carl Zeiss). For the experiments using pHrodo-labelled thymocytes, before microscopic or flow cytometric analyses, the cells were washed and resuspended in basic buffer (pH 8.8) to quench the fluorescence of non-phagocytized pHrodo-labelled ACs. For the experiments using alveolar or peritoneal macrophages, staining with anti-F4/80 and/or anti-CD11b was used to define the macrophage populations for the flow cytometric analyses. For the in vivo phagocytosis, pHrodo-labelled AC were injected intraperitoneally, and the cells were collected at different times, followed by staining with anti-F4/80 and anti-CD11b and analysed by flow cytometry. In the experiments involving annexin V or MFG-E8 as a blocking agent, AC were preincubated with 50 μg ml −1 annexin V (BD Pharmingen) or 20 μg ml −1 MFG-E8 (R&D) for 10 min at 37 °C before adding to the phagocytes. In the experiments using liposome-coated beads, the beads were added to phagocytes for 30 or 60 min at 37 °C, followed by three washes with PBS, fixation and analysis using confocal microscopy. Where indicated, F-actin was visualized using Alexa Fluor 568-conjugated phalloidin. Flow cytometry Alexa Fluor 488-conjugated anti-CD300f Ab diluted 1:200 was used to examine the expression of CD300f on the cell surface. Alexa Fluor 488-conjugated goat IgG diluted 1:200 was used as an isotype control. Cells were stained with antibodies for 30 min at 4 °C, washed and analysed by flow cytometry. For receptor-binding analysis, 1 × 10 6 AC were incubated with 5 μg ml −1 anti-mouse CD16/CD32 for Fc receptors blocking and then incubated with 100 μg ml −1 chimeric proteins: CD300f WT/Fc, CD300f D117A/Fc or LAIR-1 R65K/Fc at RT for 45 min, followed by staining with FITC-conjugated anti-human IgG Fc-gamma fragment-specific Ab (at a dilution of 1:100) for 15 min. Cells were washed with 2% FBS in PBS and analysed by flow cytometry. For phagocytosis analysis, the samples were prepared as stated above. The phagocytes and AC were distinguished by forward and side scatter; and in cases of primary macrophages, the phagocytes were further gated by F4/80 + and/or CD11b + . The appearance of pHrodo or TFL-4 fluorescence in the phagocyte population was monitored as an indicator of the AC engulfment. The phagocyte cell population characterized by high fluorescence of pHrodo or TFL-4 (i.e., pHrodo high or TFL-4 high ) was regarded as the cells which engulfed the AC. Data acquisition and analysis were done using FACSort flow cytometer (BD Bioscience) with Cell Quest software (v. 3.3) and analysed using FlowJo (v. 7.6; Tree Star). Immunoprecipitation and western blot analysis 1 × 10 6 L929 or J774 cells were incubated with 5 × 10 6 AC at 4 °C for 10 min, and then transferred to 37 °C for 15 min. Cells were then lysed in ice-cold lysis buffer containing 50 mM Tris (pH 7.4), 150 mM NaCl, 5 mM EDTA, 1% NP-40, 0.5% sodium deoxycholate and protease and phosphatase inhibitors cocktail (Sigma). Cellular debris was removed by centrifugation at 10,000 g for 15 min at 4 °C. Cell lysates were precleared using 10 μl of protein G magnetic beads (Invitrogen). anti-cMyc Ab (1 μg ml −1 ) was added to the lysates and incubated overnight at 4 °C, followed by addition of 20 μl protein G magnetic beads and incubation for 1 h at 4 °C. The beads were then isolated, washed four times with the lysis buffer and mixed with 30 μl SDS–PAGE loading buffer. Samples were resolved by SDS–PAGE and transferred onto PVDF membrane (Millipore). Membranes were blocked with 5% BSA (Sigma) in TBST (20 mM Tris pH 7.4, 150 mM NaCl, 0.05% Tween-20) for 1 h and then probed with antibodies (at a dilution of 1:1,000) indicated in the text. HRP-conjugated secondary antibodies (at a dilution of 1:10,000) were used to detect bound antibodies. Blots were developed with West Pico SuperSignal kit (Pierce) and visualized on Hyperfilm (Amersham Biosciences). Measurement of serum autoantibodies ANA in the mouse sera were visualized using 12-well microscope slides covered with HEp-2 cells (MBL Corporation). Slides were incubated with mouse serum at the 1/200 dilution for 30 min at room temperature. After two washes of 5 min with PBS, goat anti-mouse IgG-FITC (Sigma) was added at a 1:250 dilution for 30 min at room temperature and washed with PBS for 5 min at least three times. The fluorescence of anti-nuclear antibodies was detected by a Zeiss Axio Imager Upright microscope (Carl Zeiss) with a × 20 Zeiss Plan-Neofluar objective. ANA staining intensity score was performed in a genotype-blind fashion and was based on relative fluorescence of stained nuclear and cytoplasmic material; the scale ranged from 0 to 4 arbitrary units, according to the following criteria: 0, no fluorescence; 1, very dim fluorescence; 2, dull fluorescence; 3, distinct fluorescence; and 4, high intensity fluorescence. Serum anti-dsDNA IgG levels were quantified using a mouse anti-dsDNA IgG-specific ELISA kit (Alphadiagnostic International), according to the manufacturer’s recommendations. The plates were read at 450 nm using an ELISA plate reader. Histological analysis All tissue samples were fixed in 4% paraformaldehyde and tissue sections were stained with hematoxylin and eosin. Stained sections were scanned by a ScanScope XT (Aperio Technologies). Aperio ImageScope software (v. 11) was used for digital slide image viewing and analysis. To detect complement protein and IgG deposition in the kidney, section of the snap-frozen kidney tissue were incubated with FITC-conjugated goat F(ab′) 2 fragment directed to mouse complement C3 (MP Biomedical), and FITC-conjugated goat anti-moue IgG (γ-chain specific) (Sigma). Fluorescence was detected using a Zeiss Axio Imager Upright microscope (Carl Zeiss) with a × 20 Zeiss Plan-Neofluar objective. Confocal microscopy For cellular localization of CD300f, PI(4,5)P2, PI(3,4,5)P3, p85 and activated Rac/Cdc42 during phagocytosis, cells expressing EGFP-tagged CD300f constructs, PLCδ1-PH-YFP, Btk-PH-YFP, p85α-YFP or PBD-EYFP were incubated with or without AC. In some experiments, latrunculin A (Calbiochem) was used to block actin polarization; the phagocytes were preincubated with 2 μM latrunculin for 10 min, and the drug was present during the subsequent incubation of phagocytes with AC. The cells were plated on no. 1.5 glass dishes (MatTek Corporation), fixed with 4% paraformaldehyde in PBS for 15 min at room temperature and then visualized by confocal microscopy. To label F-actin, cells were fixed as above, permeabilized with 0.4% saponin in PBS for 15 min and stained with Alexa Fluor 568-conjugated phalloidin (1:200 dilution) for 1 h. In the cases of indirect immunofluorescence staining, cells were fixed and permeabilized as described above, and then blocked with 10% BSA in PBS, followed by incubation with the primary antibodies for 1 h at room temperature. Anti-cMyc antibody was used at 1:2,000. Finally, samples were incubated for 1 h with goat anti-mouse antibody (1:25 dilution) conjugated with Alexa Fluor 647. Cells were mounted in ProLong Gold medium (Invitrogen) and visualized by a LSM 710 laser scanning confocal microscope (Zeiss) with a × 63 Zeiss Plan-Apochromat objective and analysed using LSM710 software (v. 3.2). In the live cell imaging experiments, L929 cells expressing CD300f Only-Y276-EGFP, Life-Act-RFP (F-actin indicator), PLCδ1-PH-YFP or Btk-PH-YFP were first incubated with unlabelled or TFL-4-labelled AC at 4 °C for 10 min, to allow binding of AC to L929 cells, and then transferred to the heated chamber (37 °C) on the LSM 710 confocal microscope. For CD300f clustering analysis, unlabelled AC were added to L929 cells expressing CD300f-EGFP and cultured in the heated chamber (37 °C) on the LSM 710 confocal microscope. Image acquisition was performed at an interval of 20 or 180 s for 16, 26 or 90 min, as indicated in the text. The cells were visualized as described above. In experiments investigating dynamic changes of F-actin, L929 cells coexpressing Life-Act-RFP and either CD300f Only-Y276 or CD300f Y276F were placed in the Live Cell heated chamber (Pathology Devices) and maintained at 37 °C during the imaging process. After the AC were added, red fluorescent protein (RFP) fluorescence was imaged in all three planes ( x , y and z ) at 37 °C for 40 min, at 40 s intervals, using Olympus IX81 spinning-disk confocal microscope with × 100 Olympus PlanApo objective (heated to 37 °C). Image acquisition was performed with MetaMorph software (v. 7.7.3; Molecular Devices) using the streaming function, with the following parameters: 0.5 μm z -axial dimension, 100 ms exposure per frame, 126 frames per image stack. Three-dimensional reconstruction image was done using Imaris (v. 7.4; Bitplane). Statistical analysis The statistical significance was assessed using analysis of variance with the Bonferroni post-test, or by the two-tailed unpaired Student’s t -test (GraphPad Sotware, v. 6.0). Data are presented as mean+s.e.m., unless stated otherwise. Alpha level was set to 0.05. How to cite this article: Tian, L. et al . p85α recruitment by the CD300f phosphatidylserine receptor mediates apoptotic cell clearance required for autoimmunity suppression. Nat. Commun. 5:3146 doi: 10.1038/ncomms4146 (2014).